Regulation of asymmetric cell division and polarity by Scribble is not required for humoral immunity The production of protective antibody requires effective signalling of naive B cells following encounter with antigen, and the divergence of responding B lymphocytes into distinct lineages. Polarity proteins have recently been proposed as important mediators of both the initial B cell response, and potentially of asymmetric cell division. Here we show that, although polarity proteins of the Scribble complex, Scribble, Dlg1 and Lgl1, are expressed and polarized during early B cell activation, their deficiency has no effect on the in vivo outcome of immunization or challenge with influenza infection. Furthermore, we find a striking correlation in the differentiation outcome of daughters of single founder B cells in vitro . Taken together, our results indicate that B cell differentiation does not require polarity proteins of the Scribble complex, and the findings do not support a role for asymmetric cell division in B cell activation and differentiation. The generation of protective antibody responses relies on the production of a number of alternative differentiation outcomes following B cell activation. This includes memory cells, isotype-switched B cells, short and long-lived antibody-secreting plasma cells, as well as B cells with high affinity for antigen, which is driven by somatic hypermutation of the B cell receptor [1] . The mechanisms by which the initial signals through the B cell receptor (BCR) lead to both activation of the cell, and triggering of diverse programs of differentiation, are not well understood. Recently, a set of polarity proteins that regulate neuronal and epithelial cell fate decisions has been implicated in B cell signalling and fate determination [2] , [3] . The Scribble complex, comprising Scribble, Discs large (Dlg) and Lethal giant larvae (Lgl), regulates signalling at cell–cell contacts such as epithelial cell junctions and neuronal synapses, and influences both immediate cellular responses to signals between the cells, and subsequent cell fate decisions [4] . An important mechanism by which the Scribble complex regulates cell fate decisions is by asymmetric cell division (ACD). ACD involves the induction and maintenance of polarity during cell division, resulting in the production of two unique daughter cells with different molecular composition. ACD has been extensively studied in Drosophila sensory organ precursor development and neuroblast differentiation. Proteins of the Scribble complex are essential regulators of ACD in these tissues, controlling the distribution and function of cell fate determinant proteins such as Numb and aPKC [5] , [6] , [7] , [8] , [9] , [10] . The mammalian roles for these proteins are consistent with Drosophila systems, as deletion of Scribble [11] , Dlg1 (ref. 12 ) or Lgl1 (ref. 13 ) in mice is lethal due to disrupted neural tube closure, craniofacial dysmorphogenesis and neuroblast ACD, respectively. Several studies have shown that T cells may also utilize the Scribble complex to control cell fate through ACD [14] , [15] , [16] , [17] . More recently, it has been suggested that B cells might also utilize the Scribble complex protein, Dlg1, in control of the B cell synapse, and undergo ACD to determine lineage commitment. Dlg1 is recruited to the B cell immunological synapse and knockdown of Dlg1 impairs synapse formation and signalling [3] . During B cell differentiation, asymmetric localization of cell fate determinants and the polarity protein, aPKC, was observed in mitotic B cells and cell doublets [2] , suggesting that ACD might have similar role to that proposed in CD8 + T cells during activation [14] , [15] , [17] . However, fixed imaging of mitotic lymphocytes and doublets does not allow for functional analysis of the effects of asymmetry on the immune response, nor for assessment of whether the asymmetry is maintained following division long enough to alter responses of daughter cells, and thus, dictate subsequent fate or function. Previous functional testing of this hypothesis has been limited to pharmaceutical inhibition of aPKC [14] , [15] , but a definitive elucidation of the potential role of polarity or ACD requires genetic testing of the effect of loss of function of mediators of polarity. Given that the Scribble complex is essential for ACD mediated by aPKC [6] , [13] , [18] , and for lymphocyte polarity [19] we undertook a genetic and functional analysis of the role of these evolutionarily conserved regulators of cell polarity and asymmetric division in B cell differentiation, and during in vivo B- and T-cell responses. These experiments provided surprisingly little support for a role for ACD regulated by internal protein gradients in B cell fate determination. We found that B cells do not display significant asymmetry in the fate of their daughters in vitro . Furthermore, mice deficient in genes important for polarity regulation do not demonstrate impaired activation and differentiation in vitro and make robust immune responses in vivo . B cells polarize Scribble proteins following activation We initially established that key Scribble and Par complex proteins previously implicated in lymphocyte ACD are expressed in naive B cells ( Fig. 1a ). We next investigated the localization of polarity complexes during B cell activation induced by antigen-specific BCR engagement. B cells were isolated from mice transgenic for hen egg lysozyme (HEL) BCR and cocultured in the presence of HEL-coated or uncoated beads, interleukin (IL)-4 and CD40 crosslinking antibody and localization of intracellular proteins measured at 5, 24 and 48 h post stimulation. Using the Scribble protein as a marker of Scribble complex localization within B cells, we demonstrated that both the microtubule organizing centre and Scribble are localized and maintained at the BCR during activation in over 80% of B cells at 24 h post stimulation ( Fig. 1b ). Thus, similar to CD8 + T cells, Scribble complex proteins are expressed in B cells, and Scribble is polarized during B cell activation, suggesting that polarity proteins may regulate B cell activation. 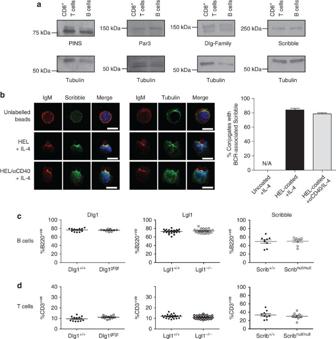Figure 1: Expression and localization of polarity proteins in B cells and function in haematopoesis. (a) Lysates were prepared from naive resting splenic B cells and CD62LhiCD8+T cells, and assayed for expression of Scribble and Par complex polarity proteins. (b) B cells were isolated from mice transgenic for HEL BCR and incubated with unlabelled beads, HEL-coated beads +IL-4 or HEL-coated beads +IL-4 and αCD40 antibody. After 24 h, cultures were cytospun onto microscope slides, fixed, permeabilized and stained to measure localization of the BCR (red), Scribble (green) and microtubule organizing centre (green). In merged images, the nucleus is labelled with 4',6-diamidino-2-phenylindole (DAPI) (blue). Images are representative of three independent experiments. White bar=10 μm. (b-right panel) B cells that formed conjugates with beads were scored for the asymmetric localization of Scribble protein at the BCR. Results are pooled from three independent experiments (Hel+IL-4=75 conjugates scored; HEL/αCD40+IL-4=70 conjugates scored). Data shown are mean±s.e.m. of three independent experiments. No conjugates were observed in cultures with unlabelled beads. Fetal livers from E13.5 to 14.5Dlggt/gt,Lgl1-/-andScribblenull/nullmice were used to reconstitute Ly5.1 (Dlg1 and Lgl1) or severe combined immunodeficiency (Scribble) mice and the proportions of (c) B cells or (d) T cells in peripheral blood measured 6–10 weeks post injection. Figure 1: Expression and localization of polarity proteins in B cells and function in haematopoesis. ( a ) Lysates were prepared from naive resting splenic B cells and CD62L hi CD8 + T cells, and assayed for expression of Scribble and Par complex polarity proteins. ( b ) B cells were isolated from mice transgenic for HEL BCR and incubated with unlabelled beads, HEL-coated beads +IL-4 or HEL-coated beads +IL-4 and αCD40 antibody. After 24 h, cultures were cytospun onto microscope slides, fixed, permeabilized and stained to measure localization of the BCR (red), Scribble (green) and microtubule organizing centre (green). In merged images, the nucleus is labelled with 4',6-diamidino-2-phenylindole (DAPI) (blue). Images are representative of three independent experiments. White bar=10 μm. ( b -right panel) B cells that formed conjugates with beads were scored for the asymmetric localization of Scribble protein at the BCR. Results are pooled from three independent experiments (Hel+IL-4=75 conjugates scored; HEL/αCD40+IL-4=70 conjugates scored). Data shown are mean±s.e.m. of three independent experiments. No conjugates were observed in cultures with unlabelled beads. Fetal livers from E13.5 to 14.5 Dlg gt/gt , Lgl1 -/- and Scribble null/null mice were used to reconstitute Ly5.1 (Dlg1 and Lgl1) or severe combined immunodeficiency (Scribble) mice and the proportions of ( c ) B cells or ( d ) T cells in peripheral blood measured 6–10 weeks post injection. Full size image Scribble proteins are not required for B cell responses. To further assess whether polarity proteins are critical for B cell activation and differentiation, we measured antibody responses of mice deficient for three members of the Scribble complex, Dlg1, Lgl1 and Scribble. As mice deficient for these genes die in utero or as neonates [11] , [12] , [13] , we generated fetal liver chimeras. Lethally irradiated Ly5.1 + mice or severe combined immunodeficiency mice were reconstituted with E13.5–14.5 fetal liver cells isolated from polarity-gene-deficient embryos and wild-type littermate controls. Six to ten weeks post reconstitution, peripheral blood was analysed for reconstitution efficiency by expression of donor derived Ly5.2 + B cells (B220, CD19— Fig. 1c ) and T-cell populations (CD3— Fig. 1d ). The proportion of Ly5.2+ B and T lymphocytes, was not affected by loss of Dlg1, Lgl1 or Scribble suggesting that the Scribble complex is not required for haematopoiesis. Naive B cells (>95% B220, CD19, IgM, IgD+ve, >99.9% donor derived) were isolated via density separation and magnetic negative selection and analysed for in vitro responses to treatment with anti-CD40 antibody and IL-4. Proliferation (cell number calculations from carboxyfluorescein succinimidyl ester (CFSE) division tracking dye dilution [20] ) ( Fig. 2a ), division linked differentiation to antibody-secreting cells (syndecan-1/CD138 expression, Fig. 2b ), and isotype switching to IgG1 (ref. 21 ) ( Fig. 2c ) were all normal in B cells lacking either Dlg1, Lgl1 or Scribble. B cells from all three genotypes also showed similar proliferation to wild-type cells in response to lipopolysaccharide (LPS) treatment ( Fig. 2d ), and LPS-induced differentiation to antibody-secreting cells was normal for Dlg1- and Lgl1-deficient B cells ( Fig. 2e ). In contrast, Scribble null/null B cells stimulated with LPS displayed a significant increase in CD138 + plasma cells ( Fig. 2e ). Scribble expression is important in the negative regulation of extracellular signal-regulated kinase (ERK) phosphorylation in epithelial tissue [11] , [22] , [23] , and given the strong links between the activation of this signalling pathway and LPS-induced differentiation [24] , we investigated ERK phosphorylation in Scribble null/null B cells. We found that the kinetics of ERK phosphorylation were perturbed in Scribble null/null B cells with initial normal activation in response to LPS stimulation, but much weaker phosphorylation at 5 and 24 h compared with wild-type controls ( Fig. 2f ). Not withstanding these subtle effects, these results demonstrate that Scribble is capable of modulating the sensitivity of B cells to LPS-induced signalling in vitro . 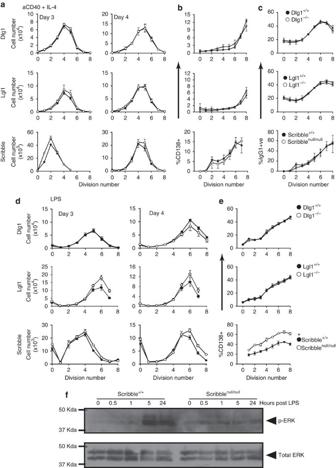Figure 2: Functional analysis of polarity-deficient B cells. Small resting splenic B cells were isolated fromDlggt/gt,Lgl1−/−andScribblenull/nullmice, CFSE labelled and stimulatedin vitrowith LPS or αCD40+IL-4, followed by measurement of proliferation (a,d), isotype switching to IgG1 (c) and differentiation to CD138+antibody-secreting cells (b,e). (f) B cells were isolated fromScribblenull/nullreconstituted mice and cultured with 20 μg ml−1LPS for the indicated time periods. Cell lysates were prepared and assayed for phosphorylation of ERK. (a–e) show representative data from three independent experiments. Data represent mean and s.e.m. of replicate cultures. *Indicates statistically significant differences as determined by two-way analysis of variance. Figure 2: Functional analysis of polarity-deficient B cells. Small resting splenic B cells were isolated from Dlg gt/gt , Lgl1 −/− and Scribble null/null mice, CFSE labelled and stimulated in vitro with LPS or αCD40+IL-4, followed by measurement of proliferation ( a , d ), isotype switching to IgG1 ( c ) and differentiation to CD138 + antibody-secreting cells ( b , e ). ( f ) B cells were isolated from Scribble null/null reconstituted mice and cultured with 20 μg ml −1 LPS for the indicated time periods. Cell lysates were prepared and assayed for phosphorylation of ERK. ( a – e ) show representative data from three independent experiments. Data represent mean and s.e.m. of replicate cultures. *Indicates statistically significant differences as determined by two-way analysis of variance. Full size image Polarized sources of stimulation and T cell help have been implicated in the induction of ACD in B cells [2] , [25] . Therefore, to mimic this scenario, we established a polarized source of CD40 stimulation by coating 4.5 μM beads with αCD40 antibody. In these cultures, microtubule organizing centres of B cells were highly polarized towards the coated beads and neighbouring cells ( Supplementary Fig S1 ). However, as with the soluble anti-CD40 ( Fig. 2a ), no differences were observed in division as measured by dilution of CFSE on days three and four ( Fig. 3a ) or by quantification of cell numbers in each division in Scribble null/null B cells ( Fig. 3b ). These cultures induce a higher rate of antibody-secreting cell commitment when compared with soluble αCD40 cultures ( Fig. 2b ), but as seen for proliferation, the production of differentiated B cells that have undergone multiple rounds of division is not dependent on expression of Scribble ( Figs 3c ). Finally, Scribble has been implicated in lymphocyte migration and we reasoned that the ability of Scribble null/null B cells to migrate and interact with each other might contribute to B lymphocyte function or ability to interact with signals from neighbouring cells. B cells were isolated from Scribble null/null mice, cultured with LPS in 8-well chamber slides lined with micro-paddocks [26] and migration tracked by live cell microscopy for 2 days. Contrary to previous findings, Scribble null/null B cells displayed no difference in migration in vitro as determined by single-cell tracking ( Figs 3e ). Furthermore, these B cells also developed uropods, which are classically observed in migrating cells ( Supplementary Fig. S2 ). 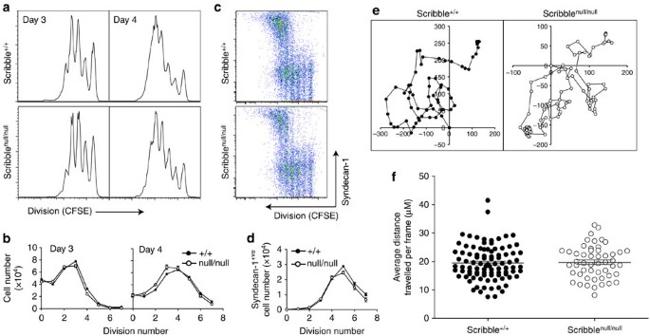Figure 3: Scribblenull/nullB cells respond to polarized stimulation and display normal migration. B cells were isolated from Scribblenull/nullreconstituted mice and wild-type littermates, CFSE labelled and cultured in the presence of αCD40 labelled 4.5 μM beads+1000 U ml−1IL-4. Proliferation was determined by dilution of CFSE (a) and quantification of cell numbers per division (b). Differentiation was determined by acquisition of syndecan-1 (CD138) expression with division (c) and quantified with relation to cell number per division (d). Data represent mean±s.e.m. of triplicate samples. (e) B cells were isolated from Scribblenull/nullreconstituted mice and wild-type littermates, and cultured in LPS for 3 days. After initial culture, B cells were seeded in micropaddocks and imaged for 48 h in an environment-controlled microscope. (e) Representative spidergrams indicating the paths of migrating B cells are shown. (f) Migration of 93 Scribble+/+and 62 Scribblenull/nullB cells was manually tracked and distance travelled calculated using ‘Metamorph’ software. The average distance travelled per frame was calculated from spidergrams. Plots represent mean±s.e.m. Data are representative from two independent experiments (e,f). Figure 3: Scribble null/null B cells respond to polarized stimulation and display normal migration. B cells were isolated from Scribble null/null reconstituted mice and wild-type littermates, CFSE labelled and cultured in the presence of αCD40 labelled 4.5 μM beads+1000 U ml −1 IL-4. Proliferation was determined by dilution of CFSE ( a ) and quantification of cell numbers per division ( b ). Differentiation was determined by acquisition of syndecan-1 (CD138) expression with division ( c ) and quantified with relation to cell number per division ( d ). Data represent mean±s.e.m. of triplicate samples. ( e ) B cells were isolated from Scribble null/null reconstituted mice and wild-type littermates, and cultured in LPS for 3 days. After initial culture, B cells were seeded in micropaddocks and imaged for 48 h in an environment-controlled microscope. ( e ) Representative spidergrams indicating the paths of migrating B cells are shown. ( f ) Migration of 93 Scribble +/+ and 62 Scribble null/null B cells was manually tracked and distance travelled calculated using ‘Metamorph’ software. The average distance travelled per frame was calculated from spidergrams. Plots represent mean±s.e.m. Data are representative from two independent experiments ( e , f ). Full size image To test in vivo B cell responses, chimeric mice were immunized with the model T-dependent antigen NP-KLH in alum followed by a secondary challenge with NP in PBS >42 days after initial challenge. All genotypes showed normal production of NP-specific low affinity antibody after primary immunization, and a progressive increase in the proportion of high affinity antibody. Additionally, on re-challenge in the absence of alum, polarity-deficient mice produced a response enriched for high affinity antibody, demonstrating that memory, somatic hypermutation and affinity maturation were intact, even in Scribble-deficient animals ( Figs 4a–f ). These data indicate that B cell development and antibody responses do not require members of the Scribble complex, with the only detectable difference being a slight increase in plasma cell differentiation after LPS treatment of Scribble-deficient B cells in vitro . 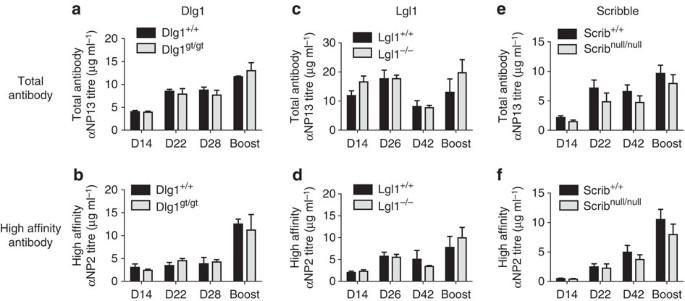Figure 4: Primary and secondary antibody responses are intact in polarity-deficient micein vivo. Dlggt/gt,Lgl1−/−andScribblenull/nullmice were challenged with NP-KLH precipitated in alum, and serum titre of total NP-specific antibody (a,cande) and high affinity NP antibody (b,dandf) measured at regular intervals. More than 40 days after primary immunization, mice were re-challenged (boosted) with NP-KLH in PBS and 10 days later serum titre was measured. Data are pooled from independent experiments, each data point represents mean±s.e.m. of serum from 3–9 mice. Figure 4: Primary and secondary antibody responses are intact in polarity-deficient mice in vivo. Dlg gt/gt , Lgl1 −/− and Scribble null/null mice were challenged with NP-KLH precipitated in alum, and serum titre of total NP-specific antibody ( a , c and e ) and high affinity NP antibody ( b , d and f ) measured at regular intervals. More than 40 days after primary immunization, mice were re-challenged (boosted) with NP-KLH in PBS and 10 days later serum titre was measured. Data are pooled from independent experiments, each data point represents mean±s.e.m. of serum from 3–9 mice. Full size image Scribble-deficient mice display intact immunity in vivo. The previous in vitro experiments revealed a phenotype only in B cells that lacked expression of Scribble. Furthermore, the Scribble protein has previously been implicated in polarization and ACD of CD8 + T-cell responses [14] , [15] , [17] , [19] , [27] . Therefore, we more closely analysed the in vivo response of Scribble-deficient mice to challenge with both NP-KLH and infection with influenza virus. Consistent with measurements of peripheral antibody titres ( Figs 4a–f ), we observed no difference in the total weight of spleens before immunization (day 14 post NP-KLH immunization—Scribble +/+ —0.108±0.015 g, Scribble null/null —0.110±0.009 g), indicating no gross change in total cell number in the spleen. Furthermore, we observed no change in the ability of Scribble-deficient mice to produce germinal centre B cells (CD19 + , IgD lo , Fas + , GL-7 + ) or germinal centre structures as determined by immunohistochemistry at days 14 and 10 post NP-KLH immunization, respectively ( Figs 5a ). Additionally, when we challenged mice with the T-cell independent antigen LPS coupled to Dinitrophenyl, serum titres of antigen-specific IgM antibody were similar to wild-type controls 10 days post immunization ( Supplementary Fig. S3 ). To test a multi-faceted immune reaction, which impacts on B cells, CD4 + and CD8 + effector and memory T-cell differentiation, we measured the response of Scribble-deficient mice to infection with HKx31 influenza virus. Primary antigen-specific CD8 + T-cell responses against the immunodominant viral epitope; nucleoprotein (NP; D b NP 366-372 ) ( Fig. 5c ) and memory responses after prior priming with the serologically distinct PR8 strain were investigated ( Fig. 5d ) (ref. 28 , 29 , 30 ). In response to both primary and secondary infection with influenza, Scribble-deficient mice produced normal proportions of antigen-specific Ly5.2 + NP + CD62L − effector CD8 + T cells at primary sites of infection such as spleen and lung ( Figs 5c ). Additionally, we observed no change in KLRG1 and IL-7 expression on Ly5.2 + NP + CD8 + T cells, indicating no bias in commitment to effector or memory precursor lineages [31] ( Fig. 4e ) or the ability to produce protective cytokines such as interferon-γ ( Fig. 4f ). Consistent with the NP-KLH immunizations, production of germinal centre B cells (Ly5.2 + B220 + CD138 - Fas + GL-7 + ) ( Fig. 5g ) was intact. The lack of differences in response to multiple antigens and routes of dose administration in vivo indicates that Scribble is not required for regulation of adaptive immunity. 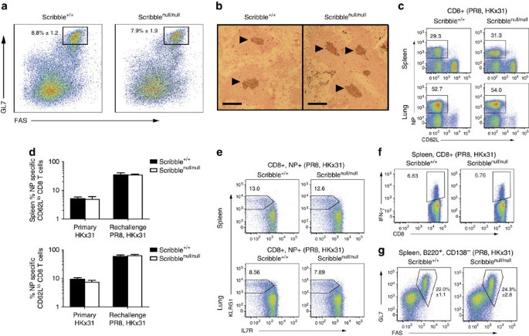Figure 5: Scribble-deficient mice mount robust immune responsesin vivo. Scribblenull/nullreconstituted mice were immunized intraperitoneally with NP-KLH precipitated on alum. (a) Ten days post NP-KLH immunization, spleens were harvested from Scribble+/+and Scribblenull/nullmice, and germinal centre B cells identified by surface expression of CD19+, IgDlo, Fas+GL-7+(n=3—data represent mean±s.e.m.). (b) Fourteen days post NP-KLH immunization, spleens were isolated, sectioned and stained to identify germinal centres (GL-7–brown) and the B cell follicle (IgD–pink). Black arrows indicate germinal centres. Scale bar shown=200 μM. Sections are representative of three mice from each genotype. (c-f) Wild-type reconstituted or Scribblenull/nullreconstituted mice were infected with influenza virus (HKx31) with or without prior priming with a heterologous influenza virus (PR8) as indicated, and virus-specific NP responses was measured 9 days later. Single-cell suspensions were prepared from either spleen or lung and analysed for Ly5.2, NP-tetramer binding and CD62L expression (c,d), as well as IL-7 and KLRG1 (e). (f) Intracellular interferon-γ staining of CD8+T cells isolated from virus-infected mice after NP-peptide re-stimulation. (g) Identification of germinal centre B cells (Ly5.2+, B220+, CD138−, FAS+, GL-7+) in virus-infected mice. (c,e–gshow representative data from pooled experiments of 3–5 mice.D=mean±s.e.m. 3–5 mice from pooled experiments). Figure 5: Scribble-deficient mice mount robust immune responses in vivo. Scribble null/null reconstituted mice were immunized intraperitoneally with NP-KLH precipitated on alum. ( a ) Ten days post NP-KLH immunization, spleens were harvested from Scribble +/+ and Scribble null/null mice, and germinal centre B cells identified by surface expression of CD19 + , IgD lo , Fas + GL-7 + ( n =3—data represent mean±s.e.m.). ( b ) Fourteen days post NP-KLH immunization, spleens were isolated, sectioned and stained to identify germinal centres (GL-7–brown) and the B cell follicle (IgD–pink). Black arrows indicate germinal centres. Scale bar shown=200 μM. Sections are representative of three mice from each genotype. ( c-f ) Wild-type reconstituted or Scribble null/null reconstituted mice were infected with influenza virus (HKx31) with or without prior priming with a heterologous influenza virus (PR8) as indicated, and virus-specific NP responses was measured 9 days later. Single-cell suspensions were prepared from either spleen or lung and analysed for Ly5.2, NP-tetramer binding and CD62L expression ( c , d ), as well as IL-7 and KLRG1 ( e ). ( f ) Intracellular interferon-γ staining of CD8 + T cells isolated from virus-infected mice after NP-peptide re-stimulation. ( g ) Identification of germinal centre B cells (Ly5.2 + , B220 + , CD138 − , FAS + , GL-7 + ) in virus-infected mice. ( c , e – g show representative data from pooled experiments of 3–5 mice. D =mean±s.e.m. 3–5 mice from pooled experiments). Full size image CD8 T-cell polarity in response to influenza antigen In light of the fact we saw no discernible impact on the response of Scribble-deficient mice to influenza infection, we decided to assess the extent of ACD in wild-type influenza responsive transgenic CD8 + T cells. To rapidly assess statistically relevant numbers we used an imaging flow cytometry-based (IFC) approach that has been validated for assessing ACD in lymphocytes [25] , [32] . This technique provides conventional flow cytometry (CFC) data with multispectral bright-field and fluorescent images, enabling assessment of ACD of all cells undergoing mitosis, and exclusion of doublet cells through strict non-biased selection, in combination with analysis of division history. As Scribble-deficient mice make a robust response to influenza infection, we used class-I restricted F5 TCR transgenic CD8 T cells that respond to influenza peptides and activated them under various conditions that should or should not induce ACD [14] , [15] , [16] , [17] . We utilized PKC-zeta (PKC-ζ) as a marker of asymmetry as it has been previously shown to be polarized during cell division during immune responses and to correlate with Scribble asymmetry [2] , [14] , [15] , [16] . Under all stimulation conditions used, we observed robust proliferation of CD8 + T cells, however, by flow cytometry we were unable to detect expected bifurcation of PKC-ζ in either live or dead cell populations [14] , [15] , [16] , [17] . We then used our IFC-based method to examine protein localization in late-stage mitotic cells that were in the process of completing the first division. Importantly, we were able to objectively identify true telophase cells about to complete first division that were clearly not conjoined doublet cells ( Fig. 6b , lower left panel) as well as anaphasic cells, where no such concerns exist ( Fig. 6b upper panel). Interestingly, we found no evidence of late mitotic cells that had apportioned either PKC-ζ or CD8 outside the limits of total protein signal variation as judged by cell trace violet (CTV) ( Figs 6c ) ( [33] , [34] ). The lack of CD8 polarization was consistent with our previous findings in response to antigen presentation by dendritic cells [15] , but the lack of PKC-ζ polarization was particularly surprising as PKC-ζ has been suggested to be polarized in several studies. In order to remain true to the activation and culture conditions used previously to examine PKC-ζ localization in B cells and T cells [2] , [14] , we added cytochalasin B for the final four hours of cultures with F5 TCR transgenic CD8 T cells activated with antigen and antigen-presenting cells. This had little or no impact on the division process in such a short window of drug exposure, but it did lead to the appearance of bi-nucleated cells in which the process of cytokinesis had failed ( Fig. 6b , right image panels). Importantly, addition of cytochalasin B significantly increased the degree of polarization of CD8, PKC-ζ, and distribution of total cellular protein (as measured by CTV distribution) ( Figs 6c ). Thus, only in the presence of cytochalasin B were we able to detect cells where CD8 and PKC-ζ polarization had exceeded normal limits set by CTV and could, therefore, genuinely be considered to have undergone ACD. These results are consistent with our in vivo analysis of immune responses in polarity deficient and a previous study using the same method, in which dividing B cells displaying asymmetric antigen localization showed equal, or symmetric, distribution of the polarity protein, PKC-ζ (ref. 25 ). 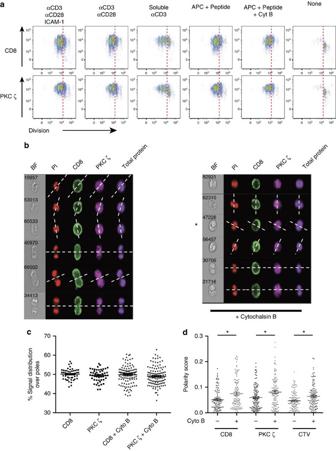Figure 6: Analysis of CD8+T-cell polarization by IFC. (a) CTV-labelled F5 CD8+T cells were activated as indicated and expression of CD8 (upper row) and PKC-ζ (lower row) assessed with division. Location of the undivided peak (red dotted line) is identified relative to unstimulated controls (b) Representative multispectral, spatially registered 40 × images of late mitotic F5 CD8+T cells in the absence (left panels) or presence (right panels) of cytochalasin B for the last 4 h of culture. Cells were stained with CD8 and PKCζ, as well as protein content and division history determined by CTV fluorescence. The plane of cytokinesis was established using the propidium iodide (PI) nuclear image (denoted by white dotted line). * Denotes example of asymmetric CD8 expression. (c,d) Polarity of each signal was calculated across daughter poles of 111 late mitotic cells entering first division and significance determined using a one-way analysis of variance. Figure 6: Analysis of CD8 + T-cell polarization by IFC. ( a ) CTV-labelled F5 CD8 + T cells were activated as indicated and expression of CD8 (upper row) and PKC-ζ (lower row) assessed with division. Location of the undivided peak (red dotted line) is identified relative to unstimulated controls ( b ) Representative multispectral, spatially registered 40 × images of late mitotic F5 CD8 + T cells in the absence (left panels) or presence (right panels) of cytochalasin B for the last 4 h of culture. Cells were stained with CD8 and PKCζ, as well as protein content and division history determined by CTV fluorescence. The plane of cytokinesis was established using the propidium iodide (PI) nuclear image (denoted by white dotted line). * Denotes example of asymmetric CD8 expression. ( c , d ) Polarity of each signal was calculated across daughter poles of 111 late mitotic cells entering first division and significance determined using a one-way analysis of variance. Full size image Stimulated B cells follow distinct lineage bias in vitro To further investigate the mechanisms driving lymphocyte fate, we established a system to track individual naive B cells and their progeny in vitro using time-lapse microscopy. Naive B cells were cultured in LPS for 24 h, and before cell division had occurred ( Supplementary Fig. S4 ), single B cells were transferred into 125 μm × 125 μm cell paddocks [26] in the presence of LPS and PE-conjugated anti-CD138 antibody. Using environment-controlled time-lapse microscopy, single cells were then imaged for 4 days. The progeny of individual founder B cells were tracked manually, and proliferation, death and differentiation to CD138-PE + plasma cells were measured. Although proliferation and differentiation varied between separate paddocks, we observed an extremely high correlation in the differentiation outcome of all progeny produced from each single founder B cell ( Fig. 7a ). For most clones, progeny were either all plasmablasts or all undifferentiated ( Fig. 7c ), suggesting a symmetrical fate inheritance from the first division of the founder B cell and arguing against a model of bifurcated differentiation. 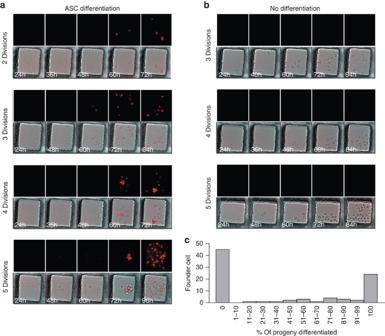Figure 7: B cell colonies from single founders adopt a uniform fate in response to LPS. Small resting splenic B cells were cultured for 24 h in LPS, then single viable B cells were transferred into 125 × 125 × 60 μm micropaddocks in the presence of LPS and αCD138-PE antibody. Cultures were imaged over another 4 days in an environment-controlled microscope. Differential interference contrast images were collected every 5 min, and PE images every 15 min. Post acquisition, 87 single B cell founders were tracked manually and the division and differentiation to CD138+antibody-secreting cells of progeny measured. Representative time-lapse images of CD138 expression (upper panels) and differential interference contrast images overlayed with CD138 expression (lower panels) for founder cells that yielded predominantly differentiated progeny (a) and undifferentiated progeny (b) are shown. Examples for founder cells that progress through 2–5 divisions are shown to illustrate that the number of divisions does not bias the differentiation commitment observed. (c) The total proportion of differentiated progeny produced by each founder cell was tracked manually and quantified. Data shown is a representative example of four independent experiments. Figure 7: B cell colonies from single founders adopt a uniform fate in response to LPS. Small resting splenic B cells were cultured for 24 h in LPS, then single viable B cells were transferred into 125 × 125 × 60 μm micropaddocks in the presence of LPS and αCD138-PE antibody. Cultures were imaged over another 4 days in an environment-controlled microscope. Differential interference contrast images were collected every 5 min, and PE images every 15 min. Post acquisition, 87 single B cell founders were tracked manually and the division and differentiation to CD138 + antibody-secreting cells of progeny measured. Representative time-lapse images of CD138 expression (upper panels) and differential interference contrast images overlayed with CD138 expression (lower panels) for founder cells that yielded predominantly differentiated progeny ( a ) and undifferentiated progeny ( b ) are shown. Examples for founder cells that progress through 2–5 divisions are shown to illustrate that the number of divisions does not bias the differentiation commitment observed. ( c ) The total proportion of differentiated progeny produced by each founder cell was tracked manually and quantified. Data shown is a representative example of four independent experiments. Full size image ACD provides an exciting possible mechanism for the production of multiple effector and memory lineages. Here we demonstrate that polarity protein networks responsible for ACD in progenitor systems are expressed in B lymphocytes and upon activation through the B cell receptor, these proteins are rapidly re-localised and asymmetrically maintained. However, despite de-regulating ERK signalling as commonly occurs with disrupted Scribble complex expression in epithelial tissue [11] , [23] , loss of Scribble complex proteins has negligible effect on the differentiation of B cells into multiple effector lineages in response to both soluble or polarized sources of stimulation in vitro . Additionally, we find that in vivo responses to primary and secondary antigen during TI and TD immunization, as well as infection with influenza virus, are not altered in the absence of Scribble complex proteins. Taken together, these data demonstrate that, although Scribble complex proteins are expressed and polarized during B cell activation, they are not necessary for effective humoral immune responses, or the provision of T cell help in germinal centres. This is surprising, and in apparent contrast to recent studies that implicate a role for Scribble complex and other polarity proteins in lymphocyte differentiation [2] , [3] , [17] . The data are compatible with recent findings that Dlg1 is not required for T-cell immune response [35] , and suggest that polarity of proteins does not necessarily predict an essential role in lymphocyte fate determination. These data, therefore, raise the question of how the extraordinary heterogeneity in lymphocyte cell fate during an immune reaction occurs and how it is controlled. The results from this study are consistent with a model whereby cell fates result from internal randomizing processes that are in constant competition [36] , [37] , rather than simple binary decisions driven by polarity protein distribution [2] . They are also consistent with a large level of external regulation of cell fate by cytokines or cell–cell interaction [25] , via varying antigen in each generation or additionally, by varying affinity for antigen [14] , [17] , [38] , [39] , [40] . Mice Mice were housed and experiments performed according to the institutional guidelines for animal experimentation of the Peter MacCallum Cancer Centre. PTPRCA-Ly5.1+ mice and severe combined immunodeficiency mice were purchased from the Walter and Eliza Hall Institute of Medical Research (Melbourne, VIC, Australia). Dlg1 +/gt [12] , Lgl1 +/- ( [13] ), FVBN/C57Bl/6-Scribble +/null -deficient or C57Bl6 Scribble +/null [11] and HEL Rag SHH/+ SHL/− Rag−/− mice (SW Hel ) [38] were bred and maintained at the Peter MacCallum Cancer Centre. Generation of chimeric mice Timed matings were established between heterozygote polarity-deficient animals. Embryos were harvested at embryonic day 14.5 and genotyped by PCR on single-cell suspensions from fetal livers. PTPRCA-Ly5.1+ or severe combined immunodeficiency recipients received two doses of 5.5 Gy administered greater than 3 h apart. 1 × 10 6 fetal liver cells were injected intravenous (i.v.). Reconstituted mice were maintained on neomycin sulphate-supplemented drinking water for 6 weeks post irradiation. Six to ten weeks post reconstitution peripheral blood was isolated from mice and stained with combinations of Ly5.2, CD3, B220, CD19, IgM and IgD to determine reconstitution efficiency. NP-KLH Immunization and enzyme-linked immunosorbent assay In vivo immunization and detection of NP-specific antibody via enzyme-linked immunosorbent assay was performed as described in Hagn et al . [41] Cell culture of mouse B cells Mouse B cells were prepared, CFSE labelled and cultured as described in Hawkins et al . [37] Cell numbers were determined by reference to fluorescence-activated cell sorting calibration beads as described in Hawkins et al . [20] B cells were typically >95% B220 + , CD19 + , IgM + , IgD + as determined by flow cytometry. Stimuli were added as follows: lipopolysaccharide derived from Salmonella typhosa (LPS, Sigma-Aldrich, St Louis, MO, USA) and anti-CD40 antibody (clone FGK4.5, WEHI) were at used at 20 μg ml −1 . IL-4 (R&D Systems, Minneapolis, USA) was added at 20 ng ml −1 . In SW HEL -transgenic B cell cultures, HEL (Sigma-Aldrich) and FGK4.5 was bound to 4.5 μM epoxy beads as described previously [42] . For in vitro differentiation studies, B cells were fixed in 2% PFA for 30 min at 4 °C and permeabilized in 0.01% Tween-20 overnight then, stained for expression of CD138 (clone 281-2, BD Pharmingen), IgM or IgG1. B cell-bead immuno-fluorescence B cell-bead conjugates were fixed at 5, 24 or 48 h post incubation and prepared as described in Oliaro et al . [15] Proteins of interest were detected with rabbit anti-Scribble (Santa Cruz, Cat. no. sc-28737), rabbit anti-tubulin (Rockland, Cat. no. 600-401-880), together with rat anti-mouse IgM (BioLegend, Cat. no. 406508) followed by the secondary antibodies (anti-rabbit-Alexa-488 and anti-rat Alexa-546, Molecular Probes). Cells were imaged using a Fluoview FV1000 confocal microscope (Olympus, Japan) with a 12.9 mW 488 nm multi-ion Argon laser, 1 mW 543 nm multi-ion green HeNe laser and 11 mW 633 nm red HeNe laser. All images were captured using a PlanApoN × 60 oil immersion objective (NA=1.42). IgM polarization to the bead was used to select conjugates for scoring of the localization of Scribble. Live cell differentiation assay B cells were isolated and cultured in LPS for 24 h using the conditions described above. After 24 h, B cells were serially diluted directly into eight-well glass chamber slides (Ibidi, Munich, Germany) with 125 × 125 × 60 μM micro-paddocks (Daniel Day, Swinburne University, Hawthorn, VIC 3122, Australia). B cells were cultured as described above with 20 μg ml −1 LPS and 80 ng ml −1 anti-CD18-PE antibody (BD Pharmingen) and imaged for 4 days in an environment-controlled microscopy chamber maintained at 37 °C and 10% CO 2. Bright-field images were acquired at 5 min intervals and PE images were acquired at 15 min time intervals. Post acquisition, proliferation (cell division), death (morphology) and differentiation (acquisition of PE+ staining) was quantified by manually. Influenza infection Viral infections and assays were performed as previously described on mice maintained on a C57Bl/6 background [30] . Briefly, mice were inoculated intranasally with 10 4.5 p.f.u. of the HKx31 (H3N2) influenza virus [28] , [43] . To measure recall responses, mice were first inoculated i.p. with 10 7 p.f.u. of the heterologous A/PR/8/34 (H1N1, PR8, Mt Sinai strain) influenza virus and then challenged intranasally with 10 4.5 p.f.u. of HKx31 6–8 weeks later [28] , [43] . Antiviral T-cell responses were enumerated by staining with PE-labelled MHC class-I tetrameric complexes specific for the nucleoprotein (D b NP 366-374 ) ( [28] , [43] ). To measure antigen-specific cytokine expression, splenocytes enriched for CD8+ T cells were stimulated in the presence of 1 μM D b NP 366-374 (ref. 44 ) peptide and 1 μg ml −1 Brefeldin A (Epicenter Biotechnologies) for 5 h. Cells were then stained for relevant surface molecules, fixed and permeabilized with the Cytofix/Cytoperm reagent (BD Biosciences) and costained for interferon-γ. Western blotting Cell lysates were prepared as follows. For polarity proteins, cells were washed twice in PBS and lysed in 100 mM NaCl, 20 mM Tris-Cl (pH 8.0), 0.5 mM EDTA and 0.5% (v/v) NP-40 in the presence of complete-Mini protease inhibitors (Roche, Mannheim, Germany). For phospho-ERK detection, cell pellets were lysed in 10% SDS, 30% Glycerol, 250 mM Tris-HCL pH 6.8 in the presence of Mini protease inhibitors and PhosStop, complete phosphatase inhibitors (Roche, Mannheim, Germany). Protein content was determined using a Bradford protein assay kit (Bio-Rad, Hercules, Ca). Lysates were boiled in either 2:1 ratio of 14 M βHYPERLINK \l "M (Sigma) to 2% bromophenol blue stock or 250 mM Tris-HCL pH 6.8, 50% glycerol W/V, 10% SDS W/V, 2.5% β-mercaptoethanol with bromophenol blue for phospho-ERK or polarity protein detection, respectively, then size-fractionated on polyacrylamide gels, and transferred to nitrocellulose membranes by electroblotting. Non-specific binding of antibodies was blocked by incubation in 5% skimmed milk and 0.05% Tween-20. For polarity proteins, the following antibodies were used: anti-Par3 (Rabbit—Upstate Biotechnology, NY, USA), Dlg-family—PSD-95 family (Upstate Biotechnology, NY, USA), PINS/GPSM2/LGN (Lifespan Biosciences, Seattle, WA, USA) and Scribble mouse monoclonal C6-D10 (ref. 44 ). Loading was determined by probing the same membrane for anti-tubulin (Cell Signalling, Danvers, MA, USA). For phospho-ERK detection, membranes were first probed with mouse anti-mouse phospho-ERK (Cell Signalling, Danvers, MA, USA Cat. no. 9106). For loading, membranes were stripped with 50 mM Tris-HCL pH 6.8, 2% SDS, 0.1 mM β-mercaptoethanol at 50 °C for 30 min, washed and membranes blocked overnight in 5% skimmed milk and 0.05% Tween-20, then re-probed with rabbit anti-mouse Total ERK (Cell Signalling, Danvers, MA, USA Cat. no. 9102). Bound antibodies were visualized by enhanced chemiluminescence (Amersham Pharmacia). Immunohistochemistry Immunohistochemistry was performed as described in Smith et al . [40] Antibodies used were unlabelled rat anti-GL-7 (ref. 40 ) and biotinylated anti-IgD (Southern Biotech, Birmingham, Alabama, USA). GL-7 was detected with anti-rat HRP (Invitrogen) and biotinylated anti-IgD with streptavidin-Alkaline-phosphatase in subsequent steps. In vitro activation of F5 CD8 T cells for analysis of ACD F5 CD8 + T cells were prepared from lymph node preps of F5.Rag1KO mice and activated with endogenous antigen-presenting cells where specified. T cells were labelled with 2.5 μM of CellTrace Violet (CTV, Invitrogen) as described previously [32] . Cells were seeded into culture at 1 million cells 1 ml −1 per well in 24-well plate then activated with different combinations of NP68 (10 nM, Mimotopes), anti-CD3 (145-2C11, eBioscience, either plate-bound at 10 μg ml −1 or in solution at 0.5 μg ml −1 ), anti-CD28 (37.51, eBioscience, plate-bound at 10 μg/ml) and recombinant ICAM1-Fc fusion (R&D Systems, plate-bound at 10 μg ml −1 ). When indicated, cytochalasin B (10 nM, SIGMA) was added for the final 4 h of the culture period as described by others [14] , [16] . Cells were cultured for up to 72 h at 37 degrees and 5% CO 2 . At point of harvest, cells were first stained for CD8a (53-6.7, FITC conjugated, eBioscience) and the LIVE/DEAD fixable near infrared dye (Invitrogen) followed by fixation for 30 min in IC fixation buffer (eBioscience). Cells were then permeabilised and stained with goat anti PKC-zeta (Santa Cruz, sc-216-G) and an AF647 labelled donkey anti-goat secondary (Invitrogen). Flow cytometry For CFC analysis, cells were stained with 7-Aminoactinomycin D and run on a 3 laser, 8 detector CANTO-II (BD). Analysis was performed in flowJo (Tree Star, USA) by gating on singlet lymphocytes (FSC/SSC gate then FSC-A/FSC-W gate) and then live cells based on LIVE/DEAD fixable near infrared dye signal exclusion. For IFC analysis the optimum harvest window was established by measuring commitment to cycling and first division using CTV dilution, 7-AAD and Ki-67 ( Supplementary Fig. S5 ). Cells were stained as for CFC but then labelled with propidium iodide (1 μg ml −1 ) and acquired on a fully calibrated ImageStream X (ISx, Amnis, USA) system as described previously using × 40 magnification [32] , [46] ). IFC analysis was performed using IDEAS software (Amnis) and Image J (v1.43, NIH, USA) as described previously [25] , [32] . Briefly, IDEAS was used to identify live mitotic cells with a known divisional history based on CTV signal dilution, bright-field and nuclear imagery, and up to nine objective pixel intensity-based features [32] . Multispectral images of CD8, PKC-zeta and CTV were the exported for each fully validated mitotic image and analysed in Image J for signal distribution (% of total) across the plane of cytokinesis [25] , [32] ( Supplementary Fig. S6 ). Polarity index was calculated using the following equation: (Square root ((%-50) squared)))/50. The threshold for asymmetry was determined using the internal control of the total protein signal as defined by CTV binding to amine groups to account for the limits of inherent protein asymmetry [33] , [34] , as well as any potential issues with imaging cells in flow [32] . How to cite this article: Hawkins E. D. et al . Regulation of asymmetric cell division and polarity by Scribble is not required for humoral immunity. Nat. Commun. 4:1801 doi: 10.1038/ncomms2796 (2013).